A central circadian oscillator confers defense heterosis in hybrids without growth vigor costs Plant immunity frequently incurs growth penalties, which known as the trade-off between immunity and growth. Heterosis, the phenotypic superiority of a hybrid over its parents, has been demonstrated for many traits but rarely for disease resistance. Here, we report that the central circadian oscillator, CCA1 , confers heterosis for bacterial defense in hybrids without growth vigor costs, and it even significantly enhances the growth heterosis of hybrids under pathogen infection. The genetic perturbation of CCA1 abrogated heterosis for both defense and growth in hybrids. Upon pathogen attack, the expression of CCA1 in F 1 hybrids is precisely modulated at different time points during the day by its rhythmic histone modifications. Before dawn of the first infection day, epigenetic activation of CCA1 promotes an elevation of salicylic acid accumulation in hybrids, enabling heterosis for defense. During the middle of every infection day, diurnal epigenetic repression of CCA1 leads to rhythmically increased chlorophyll synthesis and starch metabolism in hybrids, effectively eliminating the immunity-growth heterosis trade-offs in hybrids. Hybrids often show phenotypic superiority for many traits, such as growth rate, biomass, and stress tolerance, than their parents, a phenomenon known as hybrid vigor or heterosis [1] , which has been broadly used in crop breeding and has made an enormous contribution to world food production [2] . In contrast to the widespread utilization of heterosis in crop production over a century, our understanding of its molecular basis is still rudimentary [2] , [3] , [4] , [5] . Recent studies have identified circadian regulatory genes [6] and stress response genes [7] , [8] , [9] that contribute to growth heterosis in Arabidopsis hybrids, and enhanced salicylic acid (SA) biosynthesis contributes to bacterial defense heterosis in Arabidopsis hybrids [10] . Another study reported that a single overdominant gene, SINGLE FLOWER TRUSS , is responsible for fruit yield heterosis in tomato [11] . In addition, genome-wide association studies have identified a small number of genomic loci that contribute to yield heterosis in rice hybrids [12] , [13] and growth heterosis in Arabidopsis hybrids [14] , respectively. Moreover, several studies suggesting that both transcriptional and epigenetic variations (including DNA methylation, small RNA, and histone modifications) may play a role in the molecular mechanisms of growth heterosis [3] , [4] , [9] , [15] , [16] , [17] , [18] . Despite several studies have shed light on the potential molecular mechanisms of heterosis in plants, most have focused on heterosis for growth but rarely for heterosis for disease resistance. And, most of these studies were conducted on several candidate genes or multiple biological pathways, only a few major or single genetic factors were identified that clearly contribute to heterosis. Plant diseases cause enormous yield losses and threaten global food security. The use of highly resistant cultivars can effectively control plant disease; however, mounting a defense response frequently incurs yield penalties in plants [19] , [20] , which is known as the trade-off between defense and growth or yield. The cost of resistance was first reported in the early 1960s for late blight disease of potato ( Solanum tuberosum ) [21] and has since been documented in other crops and Arabidopsis [20] , [22] . For examples, utilization of resistance ( R ) genes, such as Wsm1 for wheat ( Triticum aestivum ) streak mosaic virus and RPM1 , RPS5 for resistance to Pseudomonas syringae in Arabidopsis , is associated with a mean yield reduction of 21% [23] and 5–10% [24] , respectively. In addition to R proteins, the Arabidopsis transcription factors TBF1 and WRKY45 enhance immunity but inhibit plant growth [25] , [26] . Conversely, the bHLH transcription factor HBI1 can promote plant growth but suppress immunity [27] , [28] . Plants have evolved several mechanisms to reduce the magnitude of immunity-growth trade-offs. In rice, a better balance between growth and immunity was obtained by a natural allele of the Broad-Spectrum Resistance-Digu 1 ( Bsr-d1 ) transcription factor gene [29] ; a single gene Ideal Plant Architecture 1 ( IPA1 ) [30] ; a nucleotide-binding oligomerization domain-like receptor (NLR) pair, Pyricularia - Gumei Resistant and Pyricularia - Gumei Susceptible ( PigmR and PigmS ) [31] ; or an artificial, pathogen-inducible cassette containing Nonexpressor of Pathogenesis-Related genes 1 ( NPR1 ) or snc1 ( suppressor of npr1-1, constitutive 1 ) [32] . Although the series of studies described above have explored the immunity-growth trade-offs in wild accessions of plants, whether and how higher plants reconcile defense and growth heterosis in hybrids, the two antagonistic biological processes, remained unexplored until now. This line of study is of substantial importance for agriculture, since it may provide an avenue to develop hybrids that have strong, durable disease resistance without yield penalties. In this study, we identified the central circadian oscillator, CCA1 , which confers significant heterosis for disease resistance in F 1 hybrids without growth vigor penalties upon pathogen invasion, by precisely enhancing the ability to resist disease and the growth of hybrids at different time points of a day and also on different infection days. Before dawn of the first infection day, epigenetic activation of CCA1 resulted in a higher burst of SA in F 1 hybrids than that in parents, which resulted in significant heterosis for defense in hybrids. In the middle of every infection day, diurnal epigenetic repression of CCA1 led to rhythmic enhancement of growth-related pathways in F 1 hybrids, which dramatically recovered the growth consumption caused by higher levels of defense in hybrids. By this time-scheduled regulation strategy, hybrids gain advantages from the control of circadian-mediated physiological and metabolic pathways, leading to better reallocation of limited resources to ensure significantly enhanced ability to resist disease with the least growth costs. CCA1 confers significant heterosis for defense in hybrids Our previous study identified an Arabidopsis hybrid Col-0 × Sei-0 (designated FCS) that shows significant heterosis for biotrophic bacterial defense (Fig. 1a ), which was attributed to an increase in the accumulation of SA in F 1 hybrids compared with both parents when the pathogen invaded [10] . To explore other factors involved in the control of heterosis for defense in FCS hybrids, we analyzed the promoter regions of previously identified above-high parent differentially expressed genes (DEGs) in FCS at 1, 2, and 3 days after infiltration with Pst DC3000 ( n = 1326, see Supplementary Data 1 ) [10] . Interestingly, the “evening element” (AAAATATCT) was the most significantly ( p = 2.66 × 10 −15 ) enriched motif in the promoter regions of these above-high parent DEGs. 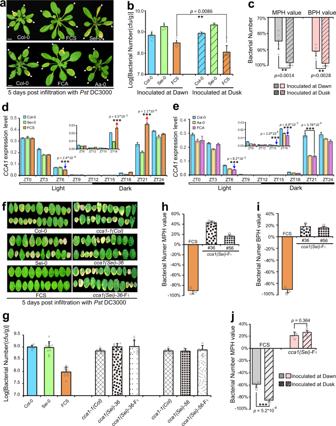Fig. 1:CCA1confers significant heterosis for defense in hybrids. aPhenotypes of F1hybrids and parents 5 dpi withPstDC3000. Arrows show the leaves inoculated with pathogen. The scale represents 1 cm.bBacterial titer (log10) of the F1hybrids and parents 5 dpi withPstDC3000 at dawn and at dusk, respectively.cMid-parent heterosis (MPH) and best-parent heterosis (BPH) values of FCS hybrids calculated by the bacterial number of 5 dpi at dawn and at dusk, respectively. Data are shown as the mean ± SD. Quantitative RT-PCR analysis of theCCA1’s expression level in the F1hybrids and parents of Col-0 × Sei-0 (d) and Col-0 × Aa-0 (e) in a 24-h period (12-h light/12-h dark cycles) starting at dawn (ZT0) withPstDC3000 infiltration. Data are shown as the mean ± SD (n= 3,nindicates biological replicates). Arrows indicate significant upregulation (red) and downregualtion (blue) ofCCA1in F1hybrids compared with that in both parents.fLeaf phenotypes of wild-type andCCA1-mutated F1hybrids and parents at 5 dpi withPstDC3000.gBacterial titer (log10) of the wild-type andCCA1-mutated F1hybrids and parents at 5 dpi withPstDC3000. MPH value (h) and BPH value (i) of wild-type andCCA1-mutated F1hybrids calculated by bacterial number at 5 dpi. Data are shown as the mean ± SD.jMPH value of wild-type andCCA1-mutated F1hybrids calculated by bacterial number (5 dpi) at dawn and dusk, respectively. Data are shown as the mean ± SD. Bacterial growth inbandgis indicated as the mean values of viable bacteria per gram of leaf tissue ± SD (n= 6,nindicates biological replicates). Both MPH and BPH values of FCS represented by the bacterial number were negative inh–jdue to the bacterial number in FCS was significantly less than that in its parents. The results inb–jare representative of three independent experiments, with measurements taken from independent samples grown and processed at different times. dpi: days post infiltration. **pvalue < 0.01; ***pvalue < 0.001 (two-tailed Student’sttest). Moreover, these evening element-containing above-high parent DEGs are significantly enriched in defense-related and circadian rhythm pathways (Supplementary Table 1 and Fig. 1 ), which imply that these DEGs are probably the targets of CCA1 or LHY [33] , [34] , and CCA1 or LHY mediated circadian clock might contribute to heterosis for bacterial defense by a significantly greater upregulation of the genes involved in defense in hybrids than both parents when the plants are attacked by a pathogen. Fig. 1: CCA1 confers significant heterosis for defense in hybrids. a Phenotypes of F 1 hybrids and parents 5 dpi with Pst DC3000. Arrows show the leaves inoculated with pathogen. The scale represents 1 cm. b Bacterial titer (log10) of the F 1 hybrids and parents 5 dpi with Pst DC3000 at dawn and at dusk, respectively. c Mid-parent heterosis (MPH) and best-parent heterosis (BPH) values of FCS hybrids calculated by the bacterial number of 5 dpi at dawn and at dusk, respectively. Data are shown as the mean ± SD. Quantitative RT-PCR analysis of the CCA1 ’s expression level in the F 1 hybrids and parents of Col-0 × Sei-0 ( d ) and Col-0 × Aa-0 ( e ) in a 24-h period (12-h light/12-h dark cycles) starting at dawn (ZT0) with Pst DC3000 infiltration. Data are shown as the mean ± SD ( n = 3, n indicates biological replicates). Arrows indicate significant upregulation (red) and downregualtion (blue) of CCA1 in F 1 hybrids compared with that in both parents. f Leaf phenotypes of wild-type and CCA1 -mutated F 1 hybrids and parents at 5 dpi with Pst DC3000. g Bacterial titer (log10) of the wild-type and CCA1 -mutated F 1 hybrids and parents at 5 dpi with Pst DC3000. MPH value ( h ) and BPH value ( i ) of wild-type and CCA1 -mutated F 1 hybrids calculated by bacterial number at 5 dpi. Data are shown as the mean ± SD. j MPH value of wild-type and CCA1 -mutated F 1 hybrids calculated by bacterial number (5 dpi) at dawn and dusk, respectively. Data are shown as the mean ± SD. Bacterial growth in b and g is indicated as the mean values of viable bacteria per gram of leaf tissue ± SD ( n = 6, n indicates biological replicates). Both MPH and BPH values of FCS represented by the bacterial number were negative in h – j due to the bacterial number in FCS was significantly less than that in its parents. The results in b – j are representative of three independent experiments, with measurements taken from independent samples grown and processed at different times. dpi: days post infiltration. ** p value < 0.01; *** p value < 0.001 (two-tailed Student’s t test). Full size image To verify this hypothesis, we first inoculated parents and hybrids with Pst DC3000 not only at the normal “dawn” infection time but also at “dusk.” We found that if Col-0, Sei-0, and their hybrids were inoculated at dusk, when infection was unexpected, significantly increased levels of susceptibility were observed in both Col-0 and Sei-0 but not in FCS. As opposed to its parents, FCS became more resistant when pathogens were inoculated at “dusk” than at “dawn” (Fig. 1b ). This result indicates that hybrids are more adaptable to unexpected infection than their parents. Calculating the mid-parent heterosis (MPH) and better-parent heterosis (BPH) values by bacterial number at 5 days post infiltration (dpi) showed that the degree of heterosis for defense was obviously higher when inoculated at “dusk” than when inoculated at “dawn” (Fig. 1c ), suggesting the involvement of the circadian clock in the regulation of heterosis for bacterial defense. Next, we tested the expression level of CCA1 in hybrids and parents grown under 12-h light/12-h dark photocycles every 3 h up to 24 h post infiltration (hpi) with or without Pst DC3000. Pst DC3000 was infiltrated at ZT0 (0 hpi, 9:00 a.m., the light is on at this time). Noticeably, when compared with that in their parents, the CCA1 ’s expression level at 21 hpi was significantly increased in FCS, while it was significantly decreased compared with mid-parent value (MPV) in another hybrid, Col-0 × Aa-0 (designated FCA), which showed no heterosis for bacterial defense (Fig. 1a, d, e ). In addition, this above-high parent pattern of expression of CCA1 in FCS only occurred when the pathogen invaded, which was not detected in the noninfiltrated condition (Fig. 1d, e and Supplementary Fig. 2 ). These results suggested that the above-high parent expression pattern of CCA1 at 21 hpi might be responsible for significant heterosis for defense in FCS hybrids, and CCA1 tends to activate defense responses before dawn of the first infection day (21 hpi) more strongly in FCS hybrids than in their parents; this time precisely precedes the peak of expression of SA biosynthetic genes at 24 hpi in the FCS hybrids [10] . To confirm the involvement of CCA1 in heterosis for defense, we generated two CRISPR/CAS9-based knockout lines of CCA1 in the Sei-0 background, each manifesting significantly decreased transcription and null translation of CCA1 (Supplementary Fig. 3 ). We obtained hybrids that were deficient in CCA1 by crossing CCA1 mutants in a Col-0 background ( cca1-1 ) with those in a Sei-0 background ( cca1(Sei)-36,56 ) and inoculated them with Pst DC3000. We noted that the CCA1 -mutated F 1 hybrids had completely lost heterosis for defense when evaluated via either phenotype or bacterial number at 5 dpi or the expression of PR1 (a marker gene that functions downstream of SA [35] ) at 24 hpi (Fig. 1f, g and Supplementary Fig. 4 ). The MPH and BPH values of the bacterial number at 5 dpi implied that the CCA1 -mutated F 1 hybrids were more susceptible than the CCA1 -mutated parents, which is opposite to the wild-type FCS phenotype (Fig. 1h, i ). Furthermore, the phenomenon that heterosis for defense was more obvious when inoculated at “dusk” than when inoculated at “dawn” disappeared in the hybrids in which CCA1 had been mutated (Fig. 1j ), implying that circadian-regulated heterosis for defense is dependent on CCA1 . Moreover, heterosis for defense was also completely abolished in the CCA1 -mutated hybrids that were generated from CRISPR/CAS9-based knockout lines in both the Col-0 and Sei-0 backgrounds (Supplementary Fig. 5 ). Unlike CCA1 , the mutation of the other two transcription factor genes, LATE ELONGATED HYPOCOTYL ( LHY ) and TIMING OF CAB2 EXPRESSION 1 ( TOC1 ), which were also involved in the core loop of eukaryotic circadian clocks [36] , [37] , did not change the degree of defense heterosis (Supplementary Figs. 6 and 7 ), and the phenomenon that heterosis for defense was more obvious when inoculated at “dusk” than when inoculated at “dawn” was also not influenced by the mutation of either LHY or TOC1 (Supplementary Fig. 8 ). These data provide strong evidence that CCA1 confers significant heterosis for defense in F 1 hybrids. 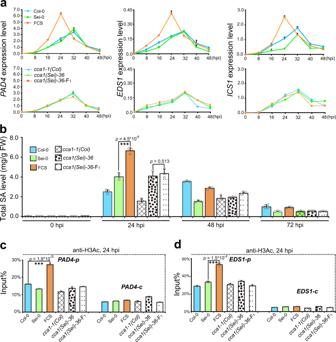Fig. 2:CCA1confers defense heterosis by enhancing salicylic acid biosynthesis in hybrids. aqPCR analyses of the expression level ofPAD4,EDS1, andICS1in Col-0 × Sei-0 andCCA1-mutated F1hybrids and parents every 8 h post infiltration (hpi) up to 48 hpi. Data are standardized for the abundance of theACTIN2transcript. Data are shown as the mean ± SD (n= 3,nindicates biological replicates).bTotal SA level in Col-0 × Sei-0 andCCA1-mutated F1hybrids and parents at 0, 24, 48, and 72 hpi withPstDC3000 inoculation. Data are shown as the mean ± SD (n= 4,nindicates biological replicates). SA salicylic acid. ChIP-qPCR analyses of promoter fragments (PAD4-pandEDS1-p) and exon fragments (PAD4-candEDS1-c) ofPAD4(c) andEDS1(d) in Col-0 × Sei-0 andCCA1-mutated F1hybrids and parents using an anti-H3Ac antibody at 24 hpi. ChIP values were normalized to their respective DNA inputs. The results are representative of three biological replicates, with measurements taken from independent samples grown and processed at different times. Data are shown as the mean ± SD (n= 3,nindicates biological replicates). ***pvalue < 0.001 (two-tailed Student’sttest). Additional F 1 hybrids and their parents ( n = 18) were selected to test the CCA1 ’s expression level at 21 hpi and calculate the MPH value of F 1 hybrids at 5 dpi (Supplementary Table 2 ). We found that in 13 of 18 hybrids (72.2%), the differential patterns of expression of CCA1 at 21 hpi were consistent with the fact that whether or not these hybrids display heterosis for defense (the cycled F 1 hybrids in Supplementary Fig. 9 ): five hybrids with an increased expression of CCA1 at 21 hpi compared with MPV show heterosis for defense (calculated by the bacterial number at 5 dpi), which is similar to the FCS hybrid, and all eight hybrids with a decreased expression of CCA1 compared with the MPV at 21 hpi show no heterosis for defense, which is similar to the FCA hybrid (Supplementary Fig. 9 ). These results imply that the above-high parent expression pattern of CCA1 in a hybrid at 21 hpi contributed to whether this hybrid exhibits heterosis for defense upon pathogen attack. Altogether, these data suggest that CCA1 is a common regulator that is essential for heterosis for defense in different Arabidopsis hybrids. CCA1 confers defense heterosis by enhancing SA biosynthesis in hybrids To further explore how CCA1 regulates heterosis for defense, we first examined the expression levels of SA biosynthetic genes in the wild-type and CCA1 -mutated parents and hybrids, including the most important SA biosynthetic gene, ICS1 [38] , [39] , the upstream transcription factor genes CBP60g , SARD1 [40] , and their upstream regulators EDS1 , PAD4 [41] , [42] , [43] . We found that the expression level of all these SA biosynthetic genes in the CCA1 -mutated hybrids did not increase significantly when compared with that in the CCA1 -mutated parents, and the 8 h earlier peak of expression in the wild-type FCS compared with that in its parents was also eliminated in the CCA1 -mutated hybrids (Fig. 2a and Supplementary Fig. 10a ). Both the significant above-high parent and the earlier expression of SA biosynthetic genes in hybrids compared with that in the parents have been shown to be essential for heterosis for defense [10] . Consistent with the pattern of expression of the SA biosynthetic genes, more SA accumulated in the wild-type hybrid of FCS than in its parents at 24 hpi ( p < 0.01, Student’s t test), which was not observed in the CCA1 -mutated hybrids (Fig. 2b ), indicating that CCA1 is an essential regulator for the above-high parent accumulation of SA in the F 1 hybrids. Fig. 2: CCA1 confers defense heterosis by enhancing salicylic acid biosynthesis in hybrids. a qPCR analyses of the expression level of PAD4 , EDS1 , and ICS1 in Col-0 × Sei-0 and CCA1 -mutated F 1 hybrids and parents every 8 h post infiltration (hpi) up to 48 hpi. Data are standardized for the abundance of the ACTIN2 transcript. Data are shown as the mean ± SD ( n = 3, n indicates biological replicates). b Total SA level in Col-0 × Sei-0 and CCA1 -mutated F 1 hybrids and parents at 0, 24, 48, and 72 hpi with Pst DC3000 inoculation. Data are shown as the mean ± SD ( n = 4, n indicates biological replicates). SA salicylic acid. ChIP-qPCR analyses of promoter fragments ( PAD4-p and EDS1-p ) and exon fragments ( PAD4-c and EDS1-c ) of PAD4 ( c ) and EDS1 ( d ) in Col-0 × Sei-0 and CCA1 -mutated F 1 hybrids and parents using an anti-H3Ac antibody at 24 hpi. ChIP values were normalized to their respective DNA inputs. The results are representative of three biological replicates, with measurements taken from independent samples grown and processed at different times. Data are shown as the mean ± SD ( n = 3, n indicates biological replicates). *** p value < 0.001 (two-tailed Student’s t test). Full size image It is notable that the mutation of CCA1 specifically affects the above-high parent expression of SA biosynthetic genes and SA accumulation in F 1 hybrid, but does not block SA biosynthesis itself in parents. Given that the increased histone H3 acetylation (H3Ac) level of key SA biosynthetic genes correlates closely with their above-high parent expression in infected hybrids [10] , we investigated the levels of H3Ac of key SA biosynthetic genes in CCA1 -mutated and wild-type parents and hybrids. We found that the levels of H3Ac at the promoter regions of the genes tested were significantly increased in FCS relative to those in both parents at 24 hpi, but there was no difference in the levels of H3Ac between the CCA1 -mutated F 1 hybrids and their parents for all four genes ( PAD4 , EDS1 , CBP60g , and SARD1 ) that are essential for SA biosynthesis (Fig. 2c, d and Supplementary Fig. 10b, c ). Taken together, our results demonstrated that CCA1 confers heterosis for defense by specifically triggering the above-high parent expression of SA biosynthetic genes in the F 1 hybrids, possibly through the regulation of these genes’ histone modifications, such as H3Ac, which ultimately results in above-high parent accumulation of SA in hybrids. CCA1 confers defense heterosis in hybrids without growth vigor costs Importantly, with pathogen infection, the wild-type hybrids FCS with remarkable defense heterosis did not display growth vigor penalties, and still showed evident heterosis for growth, as indicated by a significantly higher fresh/dry weight of the rosette or infiltrated leaves than that of its both parents at 5 dpi (Figs. 1a and 3b and Supplementary Fig. 11 ). Even more notably, the growth heterosis of FCS became more evident under disease pressure compared with that in the noninfiltration condition (without pathogen infection): the MPH value of rosette fresh weight in hybrids increased significantly from 21.9 to 30.4% ( p value = 0.0093) after pathogen invasion, indicating that the hybrids can obviously reduce the growth consumption caused by immunity more effectively than their parents (Fig. 3c ). However, in CCA1 -mutated F 1 hybrids, both the defense and growth vigor were almost abolished compared with the CCA1 -mutated parents after pathogen inoculation (Figs. 1f, g and 3b ). Moreover, the decline of growth vigor caused by the mutation of CCA1 became more dramatic when pathogen invasion (with a 22% reduction of MPH and a 14.2% reduction of BPH) than that in noninfiltration condition (with a 5.7% reduction of MPH and a 7.5% reduction of BPH) (Fig. 3a–c ). These results indicate that the heterosis for growth in the FCS hybrids was partially dependent on CCA1 in noninfiltration condition, but totally dependent on CCA1 following pathogen invasion, and that hybrids achieved significant defense heterosis without consuming growth vigor is completely owing to CCA1 . Fig. 3: CCA1 confers defense heterosis in hybrids without growth vigor costs. a Phenotypes of the whole rosette of the CCA1 -mutated F 1 hybrids and parents at 5 days post infiltration. Arrows show the four leaves of each plant inoculated with the pathogen. The scale represents 1 cm. b , d Fresh weight of the whole rosette of wild-type and CCA1 -mutated hybrids and parents simultaneously with Pst DC3000 infiltration or not. 20-day-old (counted from the day the seedlings were transferred from MS plates to the soil) plants were infiltrated with Pst DC3000 or not infiltrated. The fresh weight of whole rosette was calculated 5 days later for both noninoculated and inoculated genotypes. Data are shown as the mean ± SD ( n = 20 plants for each genotype without Pst DC3000 infiltration, and n = 30 plants for each genotype with Pst DC3000 infiltration). c , e MPH and BPH values of wild-type and CCA1 -mutated hybrids calculated by whole rosette fresh weight at the same time without (noninfiltration) or with Pst DC3000 infiltration. Data are shown as the mean ± SD. The results in c and e are representative of three independent experiments, with measurements that were taken from independent samples grown and processed at different times. * p value < 0.05; ** p value < 0.01; and *** p value < 0.001 (two-tailed Student’s t test). Full size image Another F 1 hybrids, FCA, which crossed from Col-0 and Aa-0, also showed significant heterosis for growth after pathogen inoculation (Figs. 1 a and 3d ). Similar to that of FCS, the growth vigor of FCA became even more evident under pathogen pressure compared with that in noninfiltration condition: the MPH value of rosette fresh weight in the FCA hybrids increased significantly from 43 to 66% ( p value = 0.0016) after pathogen infection. In contrast, the mutation of CCA1 , which was mutated in both Col-0 and Aa-0 background, almost abolished the growth vigor of FCA upon pathogen invasion with a 51% reduction of both MPH and BPH, but it only significantly decreased the growth vigor of FCA in noninfiltration condition with a 19% reduction of MPH and a 23% reduction of BPH (Fig. 3e ). This indicates that CCA1 also plays an important role in the growth vigor of FCA hybrids in both noninfiltration or pathogen infection conditions and is exceptionally important under conditions of pathogen invasion. Unlike FCS, the defense ability of FCA did not differ significantly from that of its parents, and there is no evident heterosis for defense in the FCA hybrids at 5 dpi; in addition, the mutation of CCA1 maintained no heterosis for defense in FCA, which is consistent with the lack of above-high parent pattern of expression of CCA1 at 21 hpi in the FCA hybrids compared with their parents (Fig. 1e and Supplementary Figs. 2 and 12 ). Taken together, all these results suggested that CCA1 confers significant defense heterosis in hybrids without growth vigor penalties and even dramatically promotes growth heterosis in hybrids under pathogen infection. 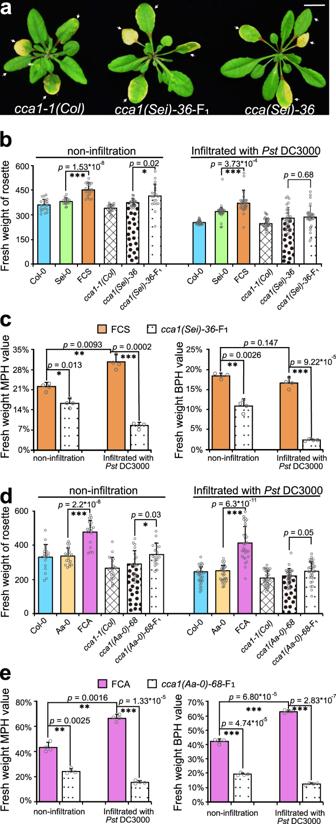Fig. 3:CCA1confers defense heterosis in hybrids without growth vigor costs. aPhenotypes of the whole rosette of theCCA1-mutated F1hybrids and parents at 5 days post infiltration. Arrows show the four leaves of each plant inoculated with the pathogen. The scale represents 1 cm.b,dFresh weight of the whole rosette of wild-type andCCA1-mutated hybrids and parents simultaneously withPstDC3000 infiltration or not. 20-day-old (counted from the day the seedlings were transferred from MS plates to the soil) plants were infiltrated withPstDC3000 or not infiltrated. The fresh weight of whole rosette was calculated 5 days later for both noninoculated and inoculated genotypes. Data are shown as the mean ± SD (n= 20 plants for each genotype withoutPstDC3000 infiltration, andn= 30 plants for each genotype withPstDC3000 infiltration).c,eMPH and BPH values of wild-type andCCA1-mutated hybrids calculated by whole rosette fresh weight at the same time without (noninfiltration) or withPstDC3000 infiltration. Data are shown as the mean ± SD. The results incandeare representative of three independent experiments, with measurements that were taken from independent samples grown and processed at different times. *pvalue < 0.05; **pvalue < 0.01; and ***pvalue < 0.001 (two-tailed Student’sttest). In addition, we calculated heterosis for growth (MPH values) by fresh and dry weight of the rosette 5 days after pathogen inoculation, and detected the CCA1 ’s expression level at 6 hpi in 14 hybrids and parents (Supplementary Table 3 ). We found that 13 F 1 hybrids (with the exception of Ca-0-F 1 ) exhibited heterosis for growth when calculated by either fresh or dry weight at 5 dpi. In addition, 9 of these 13 F 1 hybrids (69.2%, the cycled F 1 hybrids in Supplementary Fig. 13 ) displayed a below-low parent pattern of expression of CCA1 at 6 hpi (Supplementary Fig. 13 ). These results implied that the differential pattern of expression of CCA1 in hybrids at 6 hpi also contributes to whether or not these F 1 hybrids exhibit heterosis for growth. CCA1 eliminates defense-growth heterosis trade-offs in hybrids by a time-scheduled regulation strategy Having confirmed that CCA1 confers significant defense heterosis in hybrids without growth vigor costs upon pathogen invasion, we set out to explore how CCA1 reconcile heterosis for defense and for growth, the two antagonistic biological processes, without trade-offs in the hybrids. It has been reported that plants with the CCA1 mutation were significantly more susceptible to P. syringae than the wild-type [44] . Conversely, reducing the expression of CCA1 can promote the accumulation of chlorophyll and starch, which increases the growth of plants [6] , indicating that CCA1 exhibits opposite roles in plant immunity and growth. Corresponding to the opposite role of CCA1 in immunity and growth, CCA1 manifested below-low parent expression pattern of CCA1 in FCS hybrids at 6 hpi, but converse to above-high parent expression pattern of CCA1 in the FCS hybrids at 21 hpi, which is consistent with the role of CCA1 in the significantly enhancement of both defense and growth heterosis of the FCS hybrids upon pathogen invasion. In addition, CCA1 ’s expression level decreased significantly in both the FCS and FCA hybrids compared with that in their parents at ZT6 weather or not they were inoculated with Pst DC3000 (Fig. 1d, e and Supplementary Fig. 2 ). Considering that both FCS and FCA showed significantly growth heterosis and the same below-low parent expression patterns of CCA1 at ZT6 no matter inoculated with Pst DC3000 or not (Fig. 1a, d, e and Supplementary Fig. 2 ) and that plants accumulate energy and materials required for growth during the day because the light-requiring step in chlorophyll biosynthesis can be activated [45] , we speculated that CCA1 may enhance heterosis for growth in hybrids in middle of the infection day (6 hpi). In addition, considering that only FCS showed significantly heterosis for defense (Fig. 1a, f, g and Supplementary Fig. 12d ) and CCA1 showed above-high parent expression pattern only in FCS hybrids at 21 hpi that occurred specifically upon pathogen infection (Fig. 1d, e and Supplementary Fig. 2 ), we speculated that CCA1 may confer heterosis for defense before the dawn of first infection day (21 hpi), the time that precisely precedes the peak of expression of SA biosynthetic genes and the burst of SA (24 hpi). Thus, CCA1 may confer growth and defense heterosis at different time points in a day, enabling hybrids to successfully achieve significant defense heterosis without losing their growth vigor. Since the evening element-containing above-high parent DEGs in FCS were significantly enriched in starch metabolism and photosynthesis pathway, which tightly correlated with plant growth (Supplementary Fig. 1 ), we first focused on PORA and PORB , which encode protochlorophyllide oxidoreductases a and b, and mediate the only light-requiring step in chlorophyll biosynthesis [45] . The upregulation of PORA and PORB increases the content of chlorophyll a and b, which are essential for photosynthesis in higher plants [46] . We found that PORB ’s expression level was only significantly upregulated in FCS compared with that in both parents at 6 hpi, but not at 21 hpi (the same time as ZT6 and ZT21 in Fig. 1d ), and this above-high parent of PORB ’s expression pattern in FCS was completely dependent on CCA1 (Fig. 4a ). In contrast to PORB , there is no difference between FCS hybrids and their parents for PORA ’s expression at both 6 hpi and 21 hpi, and no difference between the CCA1 -mutated hybrids and parents (Supplementary Fig. 14a ). Similar to the expression of PORB , two typical genes involved in starch degradation, GWD3 and DPE1 [47] , [48] , were also significantly upregulated in FCS only at 6 hpi but not at 21 hpi and not in the CCA1 -mutated hybrids compared with those in CCA1 -mutated parents (Fig. 4b and Supplementary Fig. 14b ). We also observed that the expression level of PORB , GWD3 , and DPE1 in the CCA1 -mutated parents and hybrids were significantly higher than those in the wild-type parents and hybrids, indicating that CCA1 inhibits these growth-related genes’ expression. The above-high parent expression of PORB , GWD3 , and DPE1 corresponds to the below-low parent expression of CCA1 in FCS at 6 hpi (Fig. 1d ), which significantly reduced the inhibition of CCA1 on these growth-related genes in hybrids compare with that in parents. Fig. 4: CCA1 eliminates defense-growth heterosis trade-offs in hybrids by a time-scheduled regulation strategy. qPCR analyses of PORB ’s ( a ) and GWD3 ’s ( b ) expression level in the F 1 hybrids and parents of Col-0 × Sei-0 at 6 hpi and 21 hpi and of cca1-1(Col) × cca1(sei)-36 at 6 hpi. Data are standardized for the abundance of the ACTIN2 transcript. Data are shown as the mean ± SD ( n = 3, n indicates biological replicates). c Chlorophyll B content of inoculated leaves in the F 1 hybrids and parents of Col-0 × Sei-0 and cca1-1(Col) × cca1(sei)-36 at 6 hpi and 21 hpi. Data are shown as the mean ± SD ( n = 4, n indicates biological replicates, six leaves for each biological replicate). d Starch content in the inoculated leaves after removing soluble sugar in the F 1 hybrids and parents of Col-0 × Sei-0 and cca1-1(Col) × cca1(sei)-36 at 6 hpi and 21 hpi. Data are shown as the mean ± SD ( n = 4, n indicates biological replicates, six leaves for each biological replicate). ChIP-qPCR analyses of promoter fragments that contained the “evening element” motif ( PORB-p and GWD3-p ) and exon fragments ( PORB-c and GWD3-c ) of PORB ( e ) and GWD3 ( f ) in F 1 hybrids and their parents using an anti-CCA1 antibody at 6 hpi. ChIP values were normalized to their respective DNA inputs. The results are representative of three biological replicates with measurements taken from independent samples grown and processed at different times. Data are shown as the mean ± SD ( n = 3, n indicates biological replicates). qPCR analyses of CCA1 expression in F 1 hybrids and the parents of Col-0 × Sei-0 at 45 hpi (ZT45) ( g ) and at 30 hpi (ZT30), 54 hpi (ZT54), 78 hpi (ZT78), and 102 hpi (ZT102) ( h ). The expression level of CCA1 were shown as the mean ± SD ( n = 3, n indicates biological replicates). Data are standardized for the abundance of the ACTIN2 transcript. hpi hours post inoculation. * p value < 0.05; ** p value < 0.01; and *** p value < 0.001 (two-tailed Student’s t test). Full size image Consistent with the above-high parent expression patterns of PORB, GWD3 and DPE1 in hybrids (Fig. 4a , b and Supplementary Fig. 14b ), the content of chlorophyll b in the inoculated leaves of FCS was significantly higher than that in the leaves of both parents at 6 hpi, which was not observed at either 21 hpi or in the CCA1 -mutated hybrids (Fig. 4c ), and the content of starch in the inoculated leaves after the removal of soluble sugar was significantly lower in FCS compared with that in both parents at 6 hpi but not at 21 hpi and in CCA1 -mutated F 1 hybrids (Fig. 4d ). Altogether, these results indicated that a greater accumulation of chlorophyll and a more rapid degradation of starch occurs specifically at 6 hpi (the middle of the infection day) in hybrids, and the significant increase in the activation of growth-related pathways in the hybrids was totally dependent on CCA1 . Since the promoter of these chlorophyll biosynthetic and starch degradative genes contain CCA1 binding motif (evening element), we speculated that CCA1 contributes to the growth vigor of FCS hybrids at 6 hpi through direct binding to these genes’ promoter to regulate their differential expression between the hybrids and parents. Besides, protein level measurement also shows that CCA1 proteins were differentially expressed between the hybrids and parents at both 6 hpi and 21 hpi (Supplementary Fig. 15 ). By the ChIP experiments, we found that CCA1 was significantly enriched in the promoter regions that contained the “evening element” but not in the exon region of these starch metabolic and photosynthetic genes (Fig. 4e, f and Supplementary Figs. 14c , 16 , and 17 ), identical to the binding of CCA1 to the TOC1 ’s promoter (Supplementary Fig. 14d ) which has been previously reported [49] . These results demonstrate that CCA1 inhibits the expression of growth-related genes by directly binding to their promoters. Moreover, this enrichment was significantly less in the FCS hybrids than that in both parents for all three of these genes but not for the control gene ACTIN2 at 6 hpi (Fig. 4e, f and Supplementary Fig. 14c, e ), which is consistent with the below-low parent expression pattern of CCA1 in FCS hybrids at 6 hpi (Fig. 1d ). In addition, the enrichment of CCA1 on the promoter of these chlorophyll biosynthetic and starch degradative genes did not differ between the FCS hybrids and parents at both 3 hpi and 24 hpi, which is consistent with the lack of differential expression pattern of CCA1 between the FCS hybrids and parents at 3 hpi and 24 hpi (Fig. 1d and Supplementary Figs. 16 and 17 ). Taken together, these results show that below-low parent expression of CCA1 in hybrids at 6 hpi significantly eliminated the inhibition of CCA1 on starch metabolic and photosynthetic genes, leading to the above-high parent expression pattern of growth-related genes in hybrids. In summary, all of these results described above illustrate that when the pathogen invades, the above-high parent expression of CCA1 at 21 hpi regulates the histone modifications of SA biosynthetic genes and enhances the burst of SA at 24 hpi in the hybrids. At the meanwhile, the below-low parent expression of CCA1 at 6 hpi specifically leads to the above-high parent expression of growth-related genes and more activation of starch metabolic and photosynthetic pathway in hybrids. With this time-scheduled regulation strategy, a single gene, CCA1 , successfully confers heterosis for defense in hybrids without influencing their growth vigor, even significantly promotes growth heterosis in hybrids under pathogen invasion. CCA1 rhythmically balances defense and growth heterosis Subsequently, to illuminate whether CCA1 enhances defense heterosis of hybrids before dawn and promotes growth heterosis of hybrids in middle of the day in a diurnal manner, we verified the expression level of CCA1 in FCS hybrids and parents in the middle of day and before dawn of every infection day. We found that CCA1 returns to the mid-parent expression pattern in FCS hybrids at 24 hpi (Fig. 1d ). In addition, no significant difference in CCA1 ’s expression was detected between FCS hybrids and parents at dawn of the second infection day (45 hpi) (Fig. 4g ), accompanied by mid-parent level of SA accumulation in the FCS hybrids at 48 hpi (Fig. 2b ). Conversely, the below-low parent expression pattern of CCA1 and significantly more accumulation of chlorophyll was detected in the FCS hybrids at 30, 54, 78, and 102 hpi (the middle of 2–5 infection days) (Fig. 4h and Supplementary Fig. 18 ). Thus, the inducible above-high parent expression pattern of CCA1 before dawn specifically occurred on the first day after infection, which not only effectively promotes heterosis for defense in hybrids precisely ahead of SA burst, but also avoids growth consumption caused by constitutive activation of CCA1 at dawn for the whole infection day. Moreover, combined with rhythmically increasing the growth heterosis in the middle of every infection day, the hybrids successfully achieved remarkable defense heterosis without growth vigor penalties, and even significantly promote growth heterosis. The core loop of eukaryotic circadian clocks consists of three transcription factors: two partly redundant morning phase factors, CCA1 and LHY, and the evening phase TOC1. CCA1/LHY and TOC1 are repressors of each other’s expression [36] , [37] . Loss function of any of these core loop genes results in a short period of CCA1 ’s clock but maintains the rhythmic expression of CCA1 [44] , [49] , [50] , [51] , [52] , [53] . Besides, TOC1 , CCA1 , and LHY can also directly repress expression of the evening complex (EC) genes, such as EARLY FLOWERING 3 ( ELF3 ) and ELF4 [54] . Mutation of ELF3 or ELF4 confers the arrhythmicity of CCA1 ’s expression [50] , [55] , [56] , [57] . To further explore whether the change in the rhythmic activity of CCA1 influences the CCA1 -mediated balanced defense and growth vigor in hybrids, we generated CRISPR/CAS9-based knockout lines of LHY , TOC1 , ELF3 , and ELF4 in the Sei-0 background, and each had a significantly decreased level of transcription in the mutated lines compared with that in the wild-type (Supplementary Figs. 6 , 7 , 21 , and 22 ). By calculating the bacterial number at 5 dpi, the expression level of PR1 at 1 dpi and the fresh weight of rosette at 5 dpi in the LHY -mutated and TOC1 -mutated hybrids, we found that heterosis for both defense and growth in FCS after Pst DC3000 inoculation was not influenced by the mutation of either LHY or TOC1 (Supplementary Figs. 6 , 7 , 19 , and 20 ). Conversely, the mutation of ELF3 or ELF4 significantly decreased heterosis for defense and for growth of FCS (Supplementary Figs. 21 and 22 ). In addition, the below-low parent expression pattern of CCA1 at 6 hpi and above-high parent expression pattern of CCA1 at 21 hpi in FCS hybrids remained in both LHY and TOC1 -mutated hybrids, but was abolished by the mutation of ELF3 and ELF4 (Supplementary Fig. 23 ). These findings demonstrate that both CCA1 and its rhythmic expression are necessary for defense and growth vigor in hybrids. Expression variations of CCA1 in hybrids correlated with its altered histone modification rhythms Previous studies implied a strong correlation between diurnal histone modifications, such as H3 lysine 4 trimethylation (H3K4me3) or acetylated H3 (H3Ac) and the rhythmic expression of CCA1 [58] , [59] . To elucidate why CCA1 exhibited a below-low parent expression pattern in the FCS hybrids at 6 hpi, but conversely, showed an above-high parent expression pattern in FCS hybrids at 21 hpi, we examined the levels of these two modifications on CCA1 in hybrids and parents at 6 hpi and 21 hpi, respectively. Both H3K4me3 and H3Ac, which mark active transcription [60] , were enriched in regions that surrounded the CCA1 TSS at 6 hpi and 21 hpi, and the enrichment of these two modifications at 21 hpi was significantly higher than that at 6 hpi (Fig. 5a–e ), which was consistent with the higher expression of CCA1 at 21 hpi than at 6 hpi (Fig. 1d ). In addition, it is worth noting that both H3K4me3 and H3Ac displayed significantly lower enrichment at 6 hpi but significantly higher enrichment at 21 hpi in FCS compared with those of both parents (Fig. 5a–e ), which is consistent with the below-low parent expression pattern of CCA1 at 6 hpi and above-high parent expression pattern of CCA1 at 21 hpi in the FCS hybrids compared with those of the parents (Fig. 1d ). Taken together, these results suggest that the altered amplitude of histone modification rhythms of CCA1 is likely to be the underlying mechanism for the observed significant changes in the transcription of CCA1 between the hybrids and parents at different time points of day. Fig. 5: Expression variations of CCA1 in hybrids correlated with its altered histone modification rhythms. a Regions of CCA1 used for the ChIP-qPCR assays. ChIP-qPCR analyses of four fragments (shown at a ) of CCA1 in the wild-type F 1 hybrids and parents using an anti-H3K4me3 antibody at 6 hpi ( b ) and 21 hpi ( d ). ChIP-qPCR analyses of four fragments (shown at a ) of CCA1 in the wild-type F 1 hybrids and parents using an anti-H3Ac antibody at 6 hpi ( c ) and 21 hpi ( e ). ChIP values in b – e were normalized to their respective DNA inputs. The results are representative of three biological replicates, with measurements taken from independent samples grown and processed at different times. Data are shown as the mean ± SD ( n = 3, n indicates biological replicates). f Working model of how CCA1 coordinates enhanced heterosis for defense and for biomass in hybrids under pathogen invasion. * p value < 0.05; ** p value < 0.01; and *** p value < 0.001 (two-tailed Student’s t test). Full size image In summary, our findings revealed that a single protein, CCA1, confers significant heterosis for defense in hybrids without consuming growth vigor upon pathogen invasion, and we uncovered a novel time-scheduled mechanism for controlling heterosis for different traits. Before the dawn of first infection day, the epigenetic activation of CCA1 enhances the level of acetylated H3 for the SA biosynthetic genes and promotes a higher burst of SA in the hybrids, leading to significant heterosis for defense. In the middle of every infection day, the diurnal epigenetic repression of CCA1 leads to the rhythmic upregulation of the downstream genes that contain the “evening element” involved in photosynthesis and starch degradation and then activates chlorophyll synthesis and starch degradation, eliminating defense-growth heterosis trade-offs in hybrids, and even dramatically enhancing the growth vigor in hybrids after pathogen invasion (Fig. 5f ). Altogether, CCA1 coordinates heterosis for both defense and growth by enhancing the disease resistance ability of hybrids at the exact time that precedes the burst of SA to avoid the growth consumption caused by the constitutive activation of CCA1 at dawn of all infection day; and rhythmically improving the growth vigor of hybrids when the light-requiring step in chlorophyll biosynthesis could be activated and maintaining this growth enhancement in a diurnal manner. CCA1 conferred heterosis for defense beyond the regulation of salicylic acid In this study, we found that CCA1 confers heterosis for defense by promoting SA biosynthesis in hybrids, which is tightly associated with the enhanced H3Ac modification of SA biosynthetic genes in hybrids regulated by CCA1 (Fig. 2 ). SA is the major phytohormone produced in response to invasion by biotrophic and hemibiotrophic pathogens [35] , [61] . The production of SA leads to the upregulation of defense pathways, as well as systemic acquired resistance [62] . In this study, we found that the epigenetic activation of CCA1 before dawn in hybrids specifically occurred on the first day of infection. This precise regulation is not only effective at increasing the accumulation of SA in hybrids but it exactly precedes the burst of SA, thus avoiding the growth consumption caused by the untimely constitutive activation of CCA1 during all infection days. It also enables hybrids to initiate the strong immune response at the very early stage of pathogen invasion. This early above-high parent accumulation of SA may also improve the systemic acquired resistance of hybrids, which benefits the plants by increasing their resistance to multiple types of pathogen invasion. In addition to SA biosynthetic pathway, several studies have shown that the resistance against Pst DC3000 is controlled by the circadian clock at multiple levels, such as the opening of stomata [44] , [54] , the pattern-triggered immunity (PTI)-induced ROS burst [63] , and the regulation of immune genes induced by MAP kinases [64] . Therefore, it is worth exploring the mechanisms that underlie how CCA1 contributes to heterosis for defense through the regulation of pathways other than SA biosynthesis. Identifying the target genes of CCA1 involved in Pst DC3000 immunity, functionally characterizing these genes, and exploring their differences in expression between hybrids and parents might be a good starting point. Multiple strategies have evolved in hybrids to eliminate defense-growth heterosis trade-offs In our previous study [10] , we found that hybridization might induce a “primed state” before pathogen invasion, which is characterized by significantly enhanced H3Ac in the promoter regions of SA biosynthetic genes in hybrids. Although this enhanced H3Ac did not induce the expression of these genes ahead of pathogen attack, but it enables a more rapid and stronger activation of SA biosynthesis and defense-related genes in hybrids upon pathogen invasion. This “primed state” effectively reduces the energetic cost for higher defense ability in hybrids. Taken together, hybrids evolved multiple strategies to reduce the magnitude of defense-growth heterosis trade-offs. Firstly, before pathogen invaded, the hybrids were primed to a physiological “state of readiness,” which prepared them for a more rapid and stronger defense response and effectively reduced the fitness cost for higher defense ability in hybrids once the pathogen invaded. Secondly, upon pathogen attack, hybrids can coordinate the defense and growth heterosis at different time points in a day. This precisely enhances the defense heterosis before dawn when exactly precedes the burst of SA (24 hpi), and promotes the growth heterosis in the middle of the day when the light-requiring step in chlorophyll biosynthesis could be activated. Thirdly, hybrids eliminate the defense-growth heterosis trade-offs by maintaining epigenetic repression of CCA1 in the middle of every infection day in a diurnal manner but inducing the epigenetic activation of CCA1 at dawn specifically on the first infection day, which effectively avoids the growth consumption caused by the constitutive activation of CCA1 at dawn of all infection days. Through these three levels of smart strategies, hybrids not only achieved significantly heterosis for defense without growth vigor costs, but also even dramatically enhance growth heterosis after pathogen infection. It is worth noting that all these strategies are associated with an alteration in the histone modifications in the hybrids. Why hybrids appear to have different histone modifications from their parents is a matter that certainly merits further investigation. What is more, we noted that the expression level of CCA1 in FCA only manifested a below-low parent expression pattern at 6 hpi, but there was no differential expression of CCA1 between FCA and its parents at 21 hpi (Fig. 1e and Supplementary Fig. 2b ), which is consistent with the fact that FCA showed only significant heterosis for growth, but no evident heterosis for defense upon pathogen invasion (Figs. 1 a and 3d and Supplementary Fig. 12d ). In addition, the mutation of CCA1 only abolished the growth vigor of FCA hybrids, but it did not affect the defense heterosis of FCA hybrids (Fig. 3d, e and Supplementary Fig. 12 ). Moreover, the differentially expression of CCA1 between F 1 hybrids and parents at 21 hpi and 6 hpi contributes to whether the F 1 hybrids showed heterosis for defense and for growth when pathogen attack, respectively (Supplementary Figs. 9 and 13 ). All these results implied that CCA1 can precisely regulate growth heterosis and defense heterosis separately at 6 hpi and 21 hpi, which also benefits the coordination of CCA1 in defense and growth heterosis in different Arabidopsis hybrids. Circadian clock regulates heterosis in a special way Our results in Fig. 3 indicating the important role of CCA1 in regulating heterosis for growth without pathogen inoculation is consistent with a previous study [6] that explained the growth vigor in allotetraploids and hybrids. In addition, our study for the first time showed that upon pathogen attack, the circadian clock is also essential for heterosis for defense, and more importantly, is crucial for coordinating the trade-offs between defense and growth heterosis. These results further illustrate the important role of CCA1 in regulation of heterosis, not only under noninfection growth conditions, but also under pathogen infection. The circadian clock integrates environmental signals with internal cues to enable proper growth, development, and response to stimuli [65] . A series of studies have shown that the circadian clock is critical for plant innate immunity [54] . We found that the circadian clock regulates heterosis for defense and balances defense-growth heterosis in a singular way, which differs from that of immunity regulation. First, the role of defense of a clock gene is not associated with its specific role in the plant clock. A mutation in any of the clock genes, such as CCA1, LHY, TOC1, ELF3 , and ELF4 , conferred enhanced disease susceptibility to P. syringae despite the fact that these genes play different roles in clock precision [54] . Conversely, we found that CCA1 is the specific core loop genes that confers both defense and growth heterosis in hybrids; neither LHY nor TOC1 were involved in this progress (Figs. 1 and 3 and Supplementary Figs. 6 , 7 , 19 , and 20 ). These observations suggest that although clock genes work together to maintain clock precision, some clock genes could affect the specific output to heterosis for defense. This is the case for CCA1 , since it is the only circadian core loop oscillator that enables coordinated heterosis for both disease resistance and growth in the same hybrid. Second, in contrast to circadian-regulated immunity, the change in rhythmic activity of CCA1 caused by a clock mutation does not predict the pathogen resistance of mutants. In the diurnal light condition, small changes in the rhythmic activity of CCA1 , such as keeping the expression of CCA1 rhythmical but changing its period of expression, as caused by a LHY or TOC1 mutation, has no influence in heterosis for both defense and growth, because CCA1 maintains below-low and above-high parent expression patterns in mutated hybrids at 6 and 21 hpi, respectively (Supplementary Figs. 6 , 7 , 19 , 20 , and 23 ). However, if we abolish the rhythmic differential expression pattern of CCA1 in hybrids, such as by mutating ELF3 or ELF4 , which confers arrhythmicity and no differential expression of CCA1 between hybrids and parents (Supplementary Fig. 23 ), the growth heterosis was decreased significantly and defense heterosis was abolished in the mutated F 1 hybrids, although CCA1 still functions normally in these hybrids (Supplementary Figs. 21 – 23 ). We are still at the beginning of understanding the role that the circadian clock plays in heterosis for defense and balancing the defense-growth heterosis trade-offs. Much research remains to be done to elucidate the underlying molecular mechanisms in clock–heterosis crosstalk, including but not limited to the identification and systematic characterization of individual clock genes in the regulation of heterosis and their deployed mechanisms, and an exploration of how these clock genes orchestrate the integration of temporal information, such as when pathogen invasion, with heterosis. Implication of CCA1 -mediated balanced defense and growth heterosis in crop breeding To date, the most efficient strategy to prevent disease is to develop varieties with durable and broad-spectrum resistance [22] . The use of resistance ( R ) genes is a cost-effective strategy for the control of disease, but the easy mutation of the pathogen effectors that trigger R gene-mediated resistance leads to a quick loss of resistance and a substantial loss in yield [66] . Conversely, resistance controlled by PTI is nonrace specific and more durable because of its decreased selective pressure for pathogens to overcome host resistance [67] . In this study, we illustrated how CCA1 confers enhanced PTI in hybrids accompanied by a significant promotion of growth vigor. The N-terminus MYB-DNA binding domain of CCA1 is highly conserved among eudicots and monocots [68] , [69] , [70] . In monocotyledonous plants, CCA1 has been isolated from rice [70] and maize [68] and exhibits rhythmicity, with peak expression around dawn, which is consistent with the expression patterns of Arabidopsis CCA1 [68] , [70] . These observations imply that the functions of CCA1 in the plant clock system are highly conserved, and our newly discovered strategy about how hybrids coordinate defense and growth vigor in hybrids has substantial potential applications for crop breeding. To achieve this goal, on the one hand, we can look for a promoter that is induced by pathogen, and enhances the expression of CCA1 at specific time points to avoid deleterious effects on growth, while maintaining the normal circadian rhythm of CCA1 , to modify the expression of CCA1 in crop varieties. Alternatively, we can search for parents which have specific CCA1 alleles, on the chance that their heterozygotic state in hybrids would confer both defense and growth heterosis. Both attempts will help us to develop new crop varieties or hybrids that have strong, durable disease resistance (by PTI) and without yield penalties. In conclusion, our results provide strong evidence that CCA1 serves as the essential circadian oscillator to confer significant defense heterosis in hybrids without influencing growth vigor, which was achieved by improving the heterosis for defense and the growth of hybrids at different time points of a day when both resistance and growth are the most effective and have the least fitness cost. In addition, this was achieved and by precisely promoting defense heterosis only before the SA burst but by rhythmically enhancing growth vigor in the middle of all infection days with a diurnal manner. The novel mechanism revealed in this study is a major step forward toward uncovering how higher plants effectively confer significant defense heterosis without growth vigor penalties, and it will be of substantial interest for crop breeding by hybridization. Plant materials and growth conditions The A. thaliana accessions Aa-0 (N934) and Sei-0 (N1504) were obtained from the Nottingham A. thaliana Stock Centre (Nottingham, UK). All other accessions, Wl-0 (CS76630), Rue3.1-31 (CS76406), Ema-1 (CS76480), Koch-1 (CS76396), WalhaesB4 (CS76408), ICE107 (CS76364), NC-1 (CS76559), Bd-0 (CS76445), Ak-1 (CS76431), ICE91 (CS76362), Ba-1 (CS76441), Ca-0 (CS76459), Altai-5 (CS76433), Bay-0 (CS955), Ber (CS76448), L er -1 (CS6928), and Est (CS76485), were obtained from the Arabidopsis Biological Resource Center (Columbus, OH, USA). Crosses were performed by dissecting immature flowers before anther dehiscence and applying pollen to the exposed pistils. The F 1 hybrid lines were generated by crossing the indicated parental lines. The F 1 hybrid of cca1 and toc1 mutants were generated by crossing the homozygous and cas9-free CRISPR lines in the Sei-0 or Aa-0 background with cca1-1 and toc1-101 in the Col-0 background [44] , [56] , respectively. Plants were grown on Murashige and Skoog plates containing 1% sucrose at 22 °C under white light conditions (100 μmol m −2 s –1 ; 16 h light/8 h dark). Plants for pathogen inoculation were grown under 12-h light and 12-h dark conditions in Percival chambers (AR models) where light, temperature, and humidity could be controlled, and leaves from 3-week-old plants were used. All plants were grown at a controlled temperature (22° ± 0.2 °C) with 65% relative humidity. Light provided by Philips Alto II tubes was set at 100 µmol m −2 s −1 during the day or LL and 0 µmol m −2 s −1 at nights. Trays of plants were moved to random positions in the growth rooms every 2 days to reduce positional effects. Promoter motif analysis and Gene Ontology analysis DNA sequences from ~1000 bp upstream of the transcription start sites of the above-high parent DEGs (see Supplementary Data 1 ) between F 1 hybrid and parents [10] were extracted and scanned in the PLACE database [71] . Fisher’s exact test was used to calculate the significance of motifs in these promoters compared with the Arabidopsis genome. The p value was then adjusted by the Benjamini–Hochberg correction method to obtain the q value. Gene Ontology results were extracted from the TAIR10 gene annotation, and a functional enrichment analysis was performed at http://bioinfo.cau.edu.cn/agriGO/ . Constructs and plant transformation For the egg cell-specific promoter-controlled CRISPR/Cas9 [72] , the single guide RNA (sgRNA) sequences were selected with suggestion of CRISPR-PLANT web program ( http://crispr.hzau.edu.cn/cgi-bin/CRISPR/CRISPR ), and using pCBC-DT1T2 as the template, the sgRNA-U6-26t-U6-29p-sgRNA cassette was amplified by PCR and cloned into pHEE401. 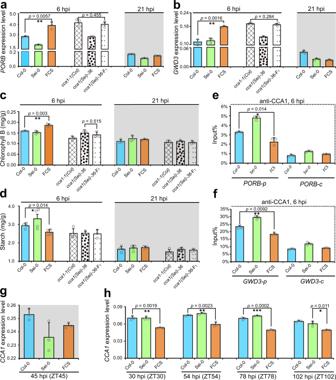Fig. 4:CCA1eliminates defense-growth heterosis trade-offs in hybrids by a time-scheduled regulation strategy. qPCR analyses ofPORB’s (a) andGWD3’s (b) expression level in the F1hybrids and parents of Col-0 × Sei-0 at 6 hpi and 21 hpi and ofcca1-1(Col)×cca1(sei)-36at 6 hpi. Data are standardized for the abundance of theACTIN2transcript. Data are shown as the mean ± SD (n= 3,nindicates biological replicates).cChlorophyll B content of inoculated leaves in the F1hybrids and parents of Col-0 × Sei-0 andcca1-1(Col)×cca1(sei)-36at 6 hpi and 21 hpi. Data are shown as the mean ± SD (n= 4,nindicates biological replicates, six leaves for each biological replicate).dStarch content in the inoculated leaves after removing soluble sugar in the F1hybrids and parents of Col-0 × Sei-0 andcca1-1(Col)×cca1(sei)-36at 6 hpi and 21 hpi. Data are shown as the mean ± SD (n= 4,nindicates biological replicates, six leaves for each biological replicate). ChIP-qPCR analyses of promoter fragments that contained the “evening element” motif (PORB-pandGWD3-p) and exon fragments (PORB-candGWD3-c) ofPORB(e) andGWD3(f) in F1hybrids and their parents using an anti-CCA1 antibody at 6 hpi. ChIP values were normalized to their respective DNA inputs. The results are representative of three biological replicates with measurements taken from independent samples grown and processed at different times. Data are shown as the mean ± SD (n= 3,nindicates biological replicates). qPCR analyses ofCCA1expression in F1hybrids and the parents of Col-0 × Sei-0 at 45 hpi (ZT45) (g) and at 30 hpi (ZT30), 54 hpi (ZT54), 78 hpi (ZT78), and 102 hpi (ZT102) (h). The expression level ofCCA1were shown as the mean ± SD (n= 3,nindicates biological replicates). Data are standardized for the abundance of theACTIN2transcript. hpi hours post inoculation. *pvalue < 0.05; **pvalue < 0.01; and ***pvalue < 0.001 (two-tailed Student’sttest). 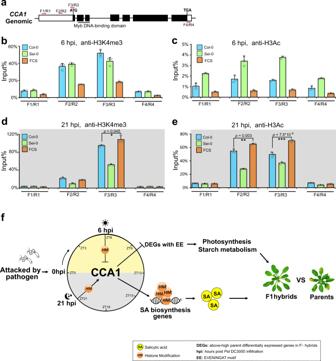Fig. 5: Expression variations ofCCA1in hybrids correlated with its altered histone modification rhythms. aRegions ofCCA1used for the ChIP-qPCR assays. ChIP-qPCR analyses of four fragments (shown ata) ofCCA1in the wild-type F1hybrids and parents using an anti-H3K4me3 antibody at 6 hpi (b) and 21 hpi (d). ChIP-qPCR analyses of four fragments (shown ata) ofCCA1in the wild-type F1hybrids and parents using an anti-H3Ac antibody at 6 hpi (c) and 21 hpi (e). ChIP values inb–ewere normalized to their respective DNA inputs. The results are representative of three biological replicates, with measurements taken from independent samples grown and processed at different times. Data are shown as the mean ± SD (n= 3,nindicates biological replicates).fWorking model of howCCA1coordinates enhanced heterosis for defense and for biomass in hybrids under pathogen invasion. *pvalue < 0.05; **pvalue < 0.01; and ***pvalue < 0.001 (two-tailed Student’sttest). The primers used for plasmid construction and for mutant screening are listed in Supplementary Table 4 . The plasmids were transformed into plants using Agrobacterium GV3101 and the floral dipping method. Transformants were selected on MS medium containing hygromycin. Western blot analysis Twelve-day-old seedlings grown in Murashige and Skoog plates that contained 1% sucrose at 22 °C under diurnal conditions (12 h light/12 h dark) were collected at 9:00 a.m. (ZT0) for Col-0, Sei-0, Aa-0, and the corresponding CCA1 -mutated lines. The CCA1 protein was detected on a 10% SDS-PAGE using a rabbit polyclonal antibody against CCA1. The CCA1-specific antibody was generated by ABclonal Biotechnology Co., Ltd. (Wuhan, China) and was used at 1:1000 dilution for western blots. The ImageJ v1.8.0_172 ( https://imagej.nih.gov/ij/ ) was used to quantify protein band intensities. RNA extraction and qRT-PCR Leaves from 3-week-old plants were infiltrated with Pst DC3000 (2 × 10 5 cfu ml –1 ) or a control and collected at different time points. At least five leaves from different plants were pooled in each sample for qRT-PCR. Leaves or 12-day-old seedlings were ground to a powder in liquid nitrogen, and total RNA was extracted using an RNeasy Plant Mini Kit (Qiagen) with an On-Column DNase I digestion treatment. Spectrophotometric and gel electrophoretic analyses were performed to detect the quality of RNA. To synthesize cDNA, 2 µg of RNA was used in the SuperScript III First-Strand Synthesis System (Invitrogen). RT-qPCR analysis (56 °C, 45 s and 45 cycles) was performed using SYBR Premix Ex Taq II mix (Takara) on an ABI7500 real-time PCR detection system (Applied Biosystems). Each experiment was repeated with three independent samples, and qRT-PCR reactions were performed in three technical replicates for each sample. The level of expression was calculated as 2 ΔΔCT and then normalized to that of A. thaliana ACTIN . All the primers used are listed in Supplementary Table 4 . Bacterial inoculation and the determination of bacterial growth Pst DC3000 was grown at 28 °C in King’s B medium (10 mg ml –1 protease peptone, 1.5 mg ml –1 K 2 HPO 4 , 15 mg ml –1 glycerol) [73] supplemented with 25 μg ml –1 rifampicin. Mature, fully expanded leaves of 3-week-old plants were infected with suspensions of bacterial cells in 10 mM MgCl 2 by pressing a 1-ml syringe (without a needle) against the abaxial side of the leaves and forcing the suspension through the stomata into the intercellular spaces. The bacterial dose was 2 × 10 5 cfu cm –2 leaf area (equivalent to OD 600 = 0.0004). Five days after inoculation, the degree of bacterial growth in plant leaves was determined by harvesting 24–32 infected leaves per sample (approximately eight plants, divided into six to eight replicates with four leaves each), and the weight of each replicate was calculated. Leaves were placed into a microcentrifuge tube containing 1 ml of 10 mM MgCl 2 and ground with a plastic pestle. This material was diluted, and 45-µl samples were spread on King’s B plates containing 25 μg ml –1 rifampicin. The plates were incubated for 2 days at 28 °C. Six to eight replicate samples per genotype were assayed to obtain means and standard deviations, which were determined from the logarithm of the number of cfu per g 2 . Determination of endogenous levels of SA Mature leaves of 3-week-old plants were infected with Pst DC3000 at a dose of 2 × 10 5 cfu cm –2 leaf area (equivalent to OD 600 = 0.0004). At 0, 24, 48, and 72 hpi, samples were collected (~0.2 g of tissue per sample, from approximately six leaves from six plants). Samples were ground in liquid nitrogen, and ~200-mg samples were mixed with 1 ml of ethyl acetate spiked with 200 ng of D 4 -SA used as an internal standard for SA. Phytohormone extraction and quantification were performed with an HPLC-MS/MS (LCMS-8040, Shimadzu, Tokyo, Japan) system. Three replicates were collected for each data point. Statistical analyses were performed using Student’s t test of the differences between the two means. Chromatin immunoprecipitation Approximately 2 g of materials was cross-linked with 1% formaldehyde in a vacuum for 35 min and were then ground to powder in liquid nitrogen. The chromatin complexes were isolated, sonicated, and then incubated with anti-AcH3 (Upstate; 06-599, 1:100 dilution), anti-H3K4me3 (Abcam; ab8580, 1:100 dilution), and anti-CCA1 (generated by ABclonal Biotechnology Co., Ltd. (Wuhan, China), rabbit polyclonal antibody, 1:100 dilution) antibodies, which were used in a 10-μl volume for immunoprecipitation. An equal amount of sample without antibody was used as a mock control. The precipitated DNA was recovered and analyzed by qPCR using specific primers listed in Supplementary Table 4 . Each ChIP value was normalized to its respective input DNA value. All ChIP-qPCR experiments were independently performed in triplicate. Chlorophyll and starch contents Mature leaves of ~3-week-old plants were infected with Pst DC3000 and were then ground to powder in liquid nitrogen. After that, chlorophyll was extracted in the dark with 1 ml of ethanol (95%) at 4 °C for 24 h. The precipitate was washed three to five times with 95% ethanol until it was completely white. The supernatant was transferred to a new tube, and the content of chlorophyll was calculated using spectrophotometric absorbance ( A ) at light wavelengths of 665 and 649 nm, with 95% ethanol as a control [74] . The chlorophyll content is shown as milligrams of chlorophyll per gram of freshly infected leaves Chlorophyll a (mg g −1 ) = 13.95 × A 665 − 6.88 × A 649 Chlorophyll b (mg g −1 ) = 24.96 × A 649 − 7.32 × A 665. The content of starch was measured from leaves inoculated with Pst DC3000 (~150 mg of fresh weight). The leaves were ground to powder in liquid nitrogen and incubated at 80 °C for 30 min in 80% ethanol to separate the soluble sugar from the starch. The total starch in each sample was then quantified using a kit from Solarbio (BC0700, China) according to the manual. Fresh/dry weight measurement Twenty-day-old soil-grown F 1 hybrids and parents were infected with Pst DC3000 at a dose of 2 × 10 5 cfu cm –2 leaf area (equivalent to OD 600 = 0.0004). Four leaves were inoculated for each plant. Five days after infiltration, the whole rosette or the infected leaves were weighed. Thirty plants and thirty replicates (four leaves for each replicate) were measured for the whole rosette and for the infected leaves, respectively. A total of 15 or 20 plants were measured for the whole rosette in noninfiltration condition. The dry weight was measured 15 days after incubation at 65 °C for the whole rosette (three plants for each replicate). Statistics and reproducibility Microsoft Excel 2019 was used to analyze qRT-PCR results and determine statistical significance based on the two-tailed Student’s t test. Statistical significance was considered when p < 0.05. The n value corresponds to the number of samples for each column, where the type of sample is indicated in the figure legends. Each experiment was repeated three times independently with similar results. Reporting summary Further information on research design is available in the Nature Research Reporting Summary linked to this article.